Bio-inspired voltage-dependent calcium channel blockers Ca 2+ influx via voltage-dependent Ca V 1/Ca V 2 channels couples electrical signals to biological responses in excitable cells. Ca V 1/Ca V 2 channel blockers have broad biotechnological and therapeutic applications. Here we report a general method for developing novel genetically encoded calcium channel blockers inspired by Rem, a small G-protein that constitutively inhibits Ca V 1/Ca V 2 channels. We show that diverse cytosolic proteins (Ca V β, 14-3-3, calmodulin and CaMKII) that bind pore-forming α 1 -subunits can be converted into calcium channel blockers with tunable selectivity, kinetics and potency, simply by anchoring them to the plasma membrane. We term this method ‘channel inactivation induced by membrane-tethering of an associated protein’ (ChIMP). ChIMP is potentially extendable to small-molecule drug discovery, as engineering FK506-binding protein into intracellular sites within Ca V 1.2-α 1C permits heterodimerization-initiated channel inhibition with rapamycin. The results reveal a universal method for developing novel calcium channel blockers that may be extended to develop probes for a broad cohort of unrelated ion channels. High-voltage-activated Ca 2+ (Ca V 1/Ca V 2) channels convert membrane electrical signals into Ca 2+ influx that drives essential processes ranging from muscle contraction to synaptic transmission [1] . Ca V 1/Ca V 2 channels are hetero-multimers comprised minimally of any one of seven pore-forming α 1 (Ca V 1.1–Ca V 1.4; Ca V 2.1–Ca V 2.3), four Ca V β (Ca V β 1 –β 4 ) and four α 2 δ (α 2 δ1–α 2 δ4) subunits in a 1:1:1 ratio [1] , [2] . Ca V 1/Ca V 2 channel inhibition is an important or potential therapy for serious disorders including hypertension, neuropathic pain, stroke, Alzheimer’s and Parkinson’s disease [3] , [4] , [5] , [6] . L-type calcium (Ca V 1.1–1.4) channels are inhibited by dihydropyridines, phenylalkylamines and benzothiazepines [7] , whereas Ca V 2.1–2.3 channels are blocked by distinct venom toxins [8] . Nevertheless, the full potential of calcium channel blocker (CCB) therapy remains unrealized due to a lack of selective and tissue-specific small-molecule inhibitors for individual Ca V 1/Ca V 2 channel types. For example, clinically used L-type CCBs do not discriminate effectively among Ca V 1.1–Ca V 1.4 isoforms [9] . As L-type channels are widely expressed, this raises significant concerns for off-target effects when targeting specific Ca V 1 isoforms for neurological disorders such as Alzheimer’s and Parkinson’s diseases [3] , [5] . Genetically encoded intracellular-acting CCBs have the potential for a high therapeutic index because they can be expressed in a locally restricted manner [2] , [10] . RGK (Rad/Rem/Rem2/Gem/Kir) GTPases are monomeric Ras-like G-proteins that powerfully inhibit all Ca V 1/Ca V 2 channels [11] , [12] , [13] . Two proof-of-concept experiments have demonstrated the potential powerful applications of RGK proteins as genetically encoded CCBs. First, local gene delivery of Gem to the atrioventricular node slowed atrioventricular nodal conduction and reduced heart rate in a porcine atrial fibrillation model [10] . Second, targeting Rem to caveolae in single cardiomyocytes permitted selective inhibition of Ca V 1.2 channels in this sub-cellular compartment [14] . The ability to inhibit Ca V 1/Ca V 2 channels in such a locally restricted manner at the whole organ or single-cell level cannot be achieved with traditional small-molecule CCBs. Ultimately, however, the potential applications of RGKs themselves as genetically encoded CCBs are limited because they do not discriminate among Ca V 1/Ca V 2 isoforms, and they have other diverse binding partners and biological functions including regulating the cytoskeleton [11] , [15] , [16] . These challenges may be overcome if it were possible to exploit the mechanism of action of RGKs to derive general principles for designing novel CCBs. Here we achieve this objective inspired by insights into how the RGK protein, Rem, inhibits Ca V 1/Ca V 2 channels. Differential tuning of Ca V 1/Ca V 2 channels by engineered Rem Wild-type Rem targets to the plasma membrane using a polybasic C terminus tail and constitutively inhibits all Ca V 1 and Ca V 2 channel isoforms. Deleting the Rem C terminus tail (Rem 265 ) ablates both membrane targeting and I Ca inhibition. We previously discovered that fusing the C1 domain from protein kinase Cγ (C1 PKC ) to Rem 1–265 enables it to be dynamically recruited to the plasma membrane with the phorbol ester, phorbol-12,13-dibutyrate (PdBu), resulting in concomitant inhibition of I Ca . A surprising, but potentially fortuitous, feature of Ca V channel inhibition by Rem 265 -C1 PKC was that it displayed apparent selectivity, being effective for Ca V 1.2 and Ca V 2.2, but inert against Ca V 2.1 and Ca V 2.3. As a prelude to investigating whether the mechanism of Rem inhibition of Ca V 1/Ca V 2 channels could be exploited to develop a general method for developing genetically encoded CCBs, we explored the possibility of tuning the selectivity and potency of PdBu-inducible Rem-based CCBs by varying the relative positioning of the C1 PKC motif in truncated Rem ( Fig. 1a ). When expressed in HEK 293 cells, all the truncated-Rem/C1 PKC fusion proteins are basally cytosolic and are rapidly recruited to the plasma membrane with PdBu ( Fig. 1b,c ). Under basal conditions, robust whole-cell currents were recorded from cells co-expressing distinct Ca V 1/Ca V 2 channel subunits (α 1 +β) and the different Rem/C1 PKC fusion constructs, enabling their selectivity and potency to be tested by adding 1 μM PdBu ( Fig. 1d–g ). Surprisingly, subtle differences in the relative position of C1 PKC in truncated Rem dramatically impacted the comparative effectiveness of the resulting protein for Ca V 2.1 and Ca V 2.2 channels. For example, CFP-Rem 1–265 -C1 PKCγ inhibited Ca V 2.2 (and Ca V 1.2) channels in response to PdBu, but was ineffective on Ca V 2.1 ( Fig. 1d,h ). In sharp contrast, simply shifting the C1 PKC motif 15 residues closer to the G-domain produced CFP-Rem 1–250 -C1 PKCγ , which permitted PdBu-induced inhibition of Ca V 2.1 (and Ca V 1.2) but was inert against Ca V 2.2 ( Fig. 1e,h ). Similarly, whereas C1 PKC -YFP-Rem 1–265 was effective for Ca V 2.2 but not Ca V 2.1 ( Fig. 1f,h ), C1 PKC -Rem 78–265 -CFP had the opposite preference, with selectivity for Ca V 2.1 over Ca V 2.2 ( Fig. 1g,h ). By contrast with the tunable selectivity for Ca V 2.2/Ca V 2.1 channels, Ca V 1.2 was uniformly sensitive to all four truncated-Rem/C1 PKC constructs. Overall, these results provide the novel observation that selectivity for distinct Ca V 2 channels can be engineered into Rem-based CCBs simply by altering the relative positioning of the inducible membrane-anchoring domain. 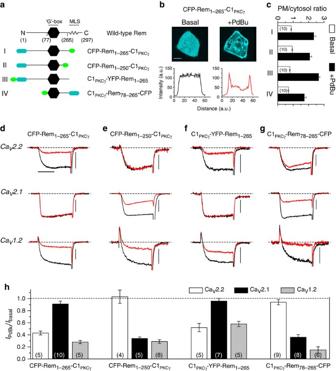Figure 1: Placement of membrane-targeting domain influences selectivity and potency of Rem-based CaV1/CaV2 channel blockers. (a) Cartoons of wild-type (wt) Rem and engineered derivatives in which an inducible membrane-targeting C1PKCdomain is placed in different positions. Wt Rem contains a guanine nucleotide-binding domain (G domain) appended by N- and C terminus extensions. The C terminus contains a polybasic sequence (MLS) that constitutively targets the protein to the plasma membrane. (b) Confocal images (top) and line scan plot (bottom) showing PdBu-induced translocation of CFP-Rem1–265-C1PKCfrom cytosol to the plasma membrane in a transfected HEK 293 cell. Scale bar, 4 μm. (c) Bar chart showing PdBu-induced increased plasma membrane to cytosol ratio for all four putative Rem-GEMIICCs. (d) Exemplar current waveforms for CaV2.2 (top), CaV2.1 (middle) and CaV1.2 (bottom) channels co-transfected with CFP-Rem1–265-C1PKCbefore (black trace) and shortly after (red trace) exposure to 1 μM PdBu. Scale bars, 400 pA, 10 ms. (e–g) Same format as (d), but with cells expressing CFP-Rem1–250-C1PKC, C1PKC-YFP-Rem1–265and C1PKC-Rem78–265-CFP, respectively. (h) Population data showing differential impact of distinct Rem-GEMIICCs on CaV2.2, CaV2.1 and CaV1.2 channels. Data are means±s.e.m. Figure 1: Placement of membrane-targeting domain influences selectivity and potency of Rem-based Ca V 1/Ca V 2 channel blockers. ( a ) Cartoons of wild-type (wt) Rem and engineered derivatives in which an inducible membrane-targeting C1 PKC domain is placed in different positions. Wt Rem contains a guanine nucleotide-binding domain (G domain) appended by N- and C terminus extensions. The C terminus contains a polybasic sequence (MLS) that constitutively targets the protein to the plasma membrane. ( b ) Confocal images (top) and line scan plot (bottom) showing PdBu-induced translocation of CFP-Rem 1–265 -C1 PKC from cytosol to the plasma membrane in a transfected HEK 293 cell. Scale bar, 4 μm. ( c ) Bar chart showing PdBu-induced increased plasma membrane to cytosol ratio for all four putative Rem-GEMIICCs. ( d ) Exemplar current waveforms for Ca V 2.2 (top), Ca V 2.1 (middle) and Ca V 1.2 (bottom) channels co-transfected with CFP-Rem 1–265 -C1 PKC before (black trace) and shortly after (red trace) exposure to 1 μM PdBu. Scale bars, 400 pA, 10 ms. ( e – g ) Same format as ( d ), but with cells expressing CFP-Rem 1–250 -C1 PKC , C1 PKC -YFP-Rem 1–265 and C1 PKC -Rem 78–265 -CFP, respectively. ( h ) Population data showing differential impact of distinct Rem-GEMIICCs on Ca V 2.2, Ca V 2.1 and Ca V 1.2 channels. Data are means±s.e.m. Full size image Conversion of auxiliary Ca V β 3 into a Ca V channel inhibitor How does Rem binding to the plasma membrane result in Ca V channel inhibition, and can this mechanism be exploited to identify a general method for developing genetically encoded CCBs? A critical clue for these questions is that in addition to membrane targeting ( Fig. 1 ), binding to auxiliary Ca V β subunits is also required for Ca V 1.2 channel inhibition by CFP-Rem 1–265 -C1 PKC [17] , [18] , [19] . Ca V βs bind the intracellular domain I–II loop of pore-forming α 1 -subunits and promote channel trafficking to the plasma membrane, as well as modulating channel activation and inactivation gating [20] . To explain the dual requirement of membrane targeting and β binding for Rem inhibition of Ca V 1.2 open probability ( P o ), we hypothesized that though cytosolic variants of Rem constitutively associate with Ca V βs in Ca V 1/Ca V 2 channel complexes, they are functionally silent, allowing the channel to gate and conduct current normally with depolarization ( Fig. 2a , top left). By contrast, membrane-targeted Rem ‘tugs’ on Ca V β and by extension, the associated α 1 -subunit I–II loop, inducing a conformational change that closes the channel pore ( Fig. 2a , top right). This allosteric model predicts it should be possible to convert the normally stimulatory Ca V β into a Ca V channel inhibitor by directly inducing its association with the plasma membrane ( Fig. 2a , bottom). We tested this idea by fusing C1 PKC directly to the C terminus of CFP-β 3 ( Fig. 2b ). CFP-β 3 -C1 PKCγ is basally cytosolic but is rapidly recruited to the plasma (and nuclear) membrane with 1 μM PdBu ( Fig. 2b , bottom left). When co-expressed with Ca V 2.2 (α 1B ), CFP-β 3 -C1 PKCγ supported robust basal Ba 2+ current ( I Ba ), signifying a retained ability to promote α 1 -subunit membrane-trafficking and modulate gating ( Fig. 2c ). Remarkably, exposure to 1 μM PdBu resulted in a gradual decrease of I Ba , peaking at 50% inhibition after 5 min ( Fig. 2c , middle). The decrease in I Ba extended across all relevant test pulse potentials, with no shift in the current density–voltage ( I – V ) relationship ( Fig. 2c , right). Importantly, control cells expressing α 1B +wild type (WT) β are not blocked by PdBu [18] ( Supplementary Fig. S1 ). Therefore, directly anchoring CFP-β 3 -C1 PKCγ to the plasma membrane translates into I Ba inhibition. This conversion of a normally stimulatory Ca V β subunit into a CCB provides strong evidence in support of the allosteric pore-closing model we propose for membrane-targeted Rem ( Fig. 2a ). 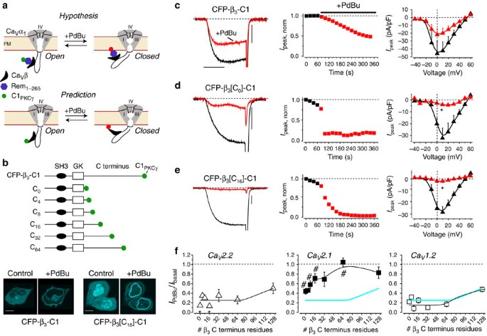Figure 2: Design of CaVβ-derived CCBs. (a) Top, hypothesis for how the dual requirement for membrane-targeting and CaVβ-binding translates into Rem inhibition of CaVchannels. Bottom, prediction for creating β-based CCBs. (b) Top, domain arrangement of CaVβ3and sites of C1PKCγplacement in the C terminus of serially truncated CaVβ3subunits. Bottom, PdBu-induced translocation of CFP-β3-C1PKCγand CFP-β3[C16]-C1PKCγfrom cytosol to plasma membrane. Scale bar, 5 μm. (c) Left, exemplar currents before (black trace) and after (red trace) exposure to PdBu in HEK 293 cell co-expressing CaV2.2α1Band CFP-β3-C1PKCγ. Scale bar, 0.5 nA, 10 ms. Middle, diary plot ofIBaamplitude before (black squares) and after (red squares) exposure to 1 μM PdBu. Right, populationI–Vcurves before (black triangles) and after (red triangles) 1 μM PdBu in cells expressing CFP-β3-C1PKCγ. Data are means±s.e.m,n=6 for each point. (d,e) Data for CFP-β3[C0]-C1PKCγand CFP-β3[C16]-C1PKCγ, respectively; same format as (c),n=6 for each point inI–Vplot. *P<0.05 compared with before PdBu data by two-tailed Student’s pairedt-test. (f) NormalizedICainhibition in HEK 293 cells expressing recombinant CaV2.2 (white triangles), CaV2.1 (black squares) or CaV1.2 (white squares) channels reconstituted with the distinct β-CCBs. Data are means±s.e.m,n=6 for each point. *significantly different from CFP-β3-C1PKCγusing one-way ANOVA and Bonferroni test. #P<0.05 compared with CaV2.2 data (blue line) by two-tailed Student’s pairedt-test. Figure 2: Design of Ca V β-derived CCBs. ( a ) Top, hypothesis for how the dual requirement for membrane-targeting and Ca V β-binding translates into Rem inhibition of Ca V channels. Bottom, prediction for creating β-based CCBs. ( b ) Top, domain arrangement of Ca V β 3 and sites of C1 PKCγ placement in the C terminus of serially truncated Ca V β 3 subunits. Bottom, PdBu-induced translocation of CFP-β 3 -C1 PKCγ and CFP-β 3 [C 16 ]-C1 PKCγ from cytosol to plasma membrane. Scale bar, 5 μm. ( c ) Left, exemplar currents before (black trace) and after (red trace) exposure to PdBu in HEK 293 cell co-expressing Ca V 2.2α 1B and CFP-β 3 -C1 PKCγ . Scale bar, 0.5 nA, 10 ms. Middle, diary plot of I Ba amplitude before (black squares) and after (red squares) exposure to 1 μM PdBu. Right, population I–V curves before (black triangles) and after (red triangles) 1 μM PdBu in cells expressing CFP-β 3 -C1 PKCγ . Data are means±s.e.m, n =6 for each point. ( d , e ) Data for CFP-β 3 [C 0 ]-C1 PKCγ and CFP-β 3 [C 16 ]-C1 PKCγ , respectively; same format as ( c ), n =6 for each point in I–V plot. * P <0.05 compared with before PdBu data by two-tailed Student’s paired t -test. ( f ) Normalized I Ca inhibition in HEK 293 cells expressing recombinant Ca V 2.2 (white triangles), Ca V 2.1 (black squares) or Ca V 1.2 (white squares) channels reconstituted with the distinct β-CCBs. Data are means±s.e.m, n =6 for each point. *significantly different from CFP-β 3 -C1 PKCγ using one-way ANOVA and Bonferroni test. # P <0.05 compared with Ca V 2.2 data (blue line) by two-tailed Student’s paired t -test. Full size image Ca V βs have a conserved core comprised of a src homology 3 (SH3) and guanylate kinase (GK)-like domains separated by a variable HOOK domain, and flanked by variable-length unstructured N- and C termini [21] , [22] , [23] . An α 1 -binding pocket in Ca V β GK binds a conserved 18-residue α 1 interaction domain in the α 1 -subunit I–II loop [21] , [22] , [23] , [24] . We hypothesized that placing C1 PKCγ closer to GK would result in a more potent, and possibly, kinetically faster β 3 -based CCB. This is because the long and presumably floppy Ca V β C terminus might be expected to introduce some slackness in the putative PdBu-induced channel conformational change ( Fig. 2a ). To test this idea we generated a series of constructs in which the relative distance between C1 PKCγ and GK was systematically varied by serial truncations of the long, unstructured β 3 C terminus ( Fig. 2b ). The most extreme case featured C1 PKCγ placed immediately downstream of GK, with no intervening β 3 C terminus sequence, generating CFP-β 3 [C 0 ]-C1 PKCγ . Cells co-expressing α 1B +CFP-β 3 [C 0 ]-C1 PKCγ displayed robust basal I Ba , and exposure to 1 μM PdBu resulted in a strong (80%), rapid-onset inhibition of current ( Fig. 2d ). A construct in which C1 PKCγ was separated from GK by 16 residues of the C terminus, CFP-β 3 [C 16 ]-C1 PKC , displayed the deepest PdBu-induced inhibition (90% inhibition at +10 mV test potential), with kinetics of onset intermediate between CFP-β 3 -C1 PKCγ and CFP-β 3 [C 0 ]-C1 PKCγ ( Fig. 2e ). Population data from experiments using distinct variable-C terminus-length constructs revealed a robust 60–90% PdBu-induced inhibition of Ca V 2.2 for β 3 -CCBs with C termini ≤64 residues, some of which were significantly different from the 50% inhibition seen with full-length β 3 ( Fig. 2f , * P <0.05 compared with CFP-β 3 -C1 PKCγ , by one-way ANOVA and Bonferroni test, n =6 for each point). Cells expressing α 1B +CFP-β 3 [C 16 ]-C1 PKC +α 2 δ-1 were similarly inhibited by PdBu, indicating that the α 2 δ-1 subunit does not prevent this effect ( Supplementary Fig. S1 ). To determine whether this mechanism of inhibition could be generalized to other Ca V channels, we also assessed the efficacy of distinct β 3 -CCBs on Ca V 2.1 and Ca V 1.2 channels ( Fig. 2f , Supplementary Figs S2 and S3 ). We found that the phenomenon was indeed evident in these other channels—for Ca V 1.2 the inhibition profile conferred by different β 3 -CCBs was similar to Ca V 2.2 ( Fig. 2f , right), whereas Ca V 2.1 displayed a solid but significantly different inhibition pattern from Ca V 2.2 ( Fig. 2f , middle, # P <0.05 compared with Ca V 2.2 inhibition, two-tailed unpaired t -test, n =6 for each point). Regarding the mechanism of inhibition of the β 3 -CCBs, we found that PdBu markedly decreased whole-cell current without affecting gating currents ( Supplementary Fig. S4 ). This suggests a selective reduction in either channel P o or single-channel conductance, with no change in the number of channels at the cell surface, similar to what we previously found for PdBu-induced Rem-based CCBs [18] . The effectiveness of membrane-targeted β 3 -CCBs in blocking Ca V 1/Ca V 2 channels was surprising given that two Ca V β isoforms, β 2a and β 2e , natively localize to the plasma membrane via their N termini, but nevertheless, yield robust I Ba when reconstituted with α 1 -subunits [25] , [26] . Moreover, artificially introducing membrane-targeting domains to N termini of cytosolic Ca V βs does not compromise their ability to reconstitute functional channels with α 1 -subunits [27] , [28] . One possibility for the discrepancy is that the polarity of the membrane-targeting domain on Ca V β is important for the impact on channel gating. We examined this idea by placing C1 PKCγ on Ca V β 3 N terminus and testing its effectiveness as a CCB. C1 PKC -β 3 -CFP reconstituted robust I Ba when co-expressed with Ca V 2.2α 1B , but exposure to PdBu had minimal impact on I Ba ( Supplementary Fig. S5 ), suggesting polarity of the membrane-targeting domain is important for β-CCB efficacy. General method for converting α 1 -binding proteins into CCBs The β 3 -CCB results are consistent with a model in which membrane-targeted Rem uses Ca V β as a ‘handle’ to alter the conformation of α 1 -subunit I–II loop in a manner that closes the channel pore. As intracellular loops and termini of Ca V 1/Ca V 2 channels ( Fig. 3a ) engage in numerous protein–protein interactions, both common and unique, we speculated that other α 1 -binding proteins might be similarly used as ‘handles’ to manipulate channel gating. If so, this would reveal a generalized principle for designing novel genetically encoded CCBs. To test this premise, we focused on three different proteins (14-3-3, Ca 2+ -calmodulin-dependent protein kinase II and calmodulin) known to bind intracellular domains of individual Ca V 1/Ca V 2 channels [29] , [30] , [31] , [32] , [33] , [34] . Wild-type 14-3-3ε binds Ca V 2.2α 1B C terminus and modulates channel inactivation properties [31] . To determine whether 14-3-3 could be converted into a small-molecule-regulated Ca V 2.2 inhibitor, we generated C1 PKCγ -mCherry-14-3-3ε, which is normally cytosolic but rapidly translocates to the plasma membrane with PdBu ( Fig. 3b ). Cells co-expressing Ca V 2.2 (α 1B +β) and C1 PKC -mCherry-14-3-3 displayed robust basal I Ba , and exposure to 1 μM PdBu caused a rapid 60% inhibition of I Ca amplitude ( Fig. 3c ). Similar results were obtained with Ca V 2.1 and Ca V 1.2, respectively, indicating that these channels also interact with 14-3-3ε ( Fig. 3c ). To our knowledge, it was not previously known that Ca V 1.2 bound 14-3-3 proteins. Replacing C1 PKCγ with an 18-residue palmitoylated membrane-targeting peptide (mem) from neuromodulin generated mem-mCherry-14-3-3ε, which constitutively targeted to the plasma membrane ( Fig. 3d ). Remarkably, mem-mCherry-14-3-3ε resulted in strong constitutive inhibition of Ca V 2.2, Ca V 2.1 and Ca V 1.2 channels across all test voltages ( Fig. 3e ). Control cells expressing mCherry-14-3-3 with Ca V 2.2 displayed neither inducible nor constitutive I Ba inhibition ( Supplementary Fig. S6 ). 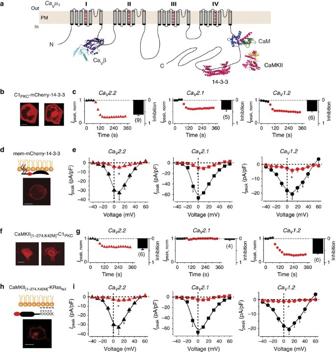Figure 3: Generalized method for generating CCBs from CaVα1-binding proteins. (a) Schematic of CaVchannel α1subunit. Four homologous domains (I–IV) each with six transmembrane segments are joined by intracellular loops and bracketed by cytoplasmic N- and C termini. Various proteins bind CaVα1intracellular domains including CaVβ, 14-3-3, CaM kinase II and calmodulin. (b) Confocal images showing PdBu-induced translocation of C1PKCγ-mCherry-14-3-3 from the cytosol to the plasma membrane. Scale bar, 4 μm. (c) Diary plots and population bar charts showing PdBu-induced inhibition of CaV2.2, CaV2.1, and CaV1.2 channels co-expressed with C1PKCγ-mCherry-14-3-3. Data are means±s.e.m. (d) Schematic and confocal image showing constitutive membrane targeting of mem-mCherry-14-3-3. Scale bar, 5 μm. (e) PopulationI–Vcurves showing constitutive inhibition by mem-mCherry-14-3-3 of CaV2.2 (black triangles, red triangles), CaV2.1 (black squares, red squares) and CaV1.2 (black circles, red circles) channels. Data are means±s.e.m,n=5 for each point. *P<0.05 compared with control data by two-tailed Student’s pairedt-test. (f) PdBu-induced translocation of mCherry-CaMKII1–274,K42M-C1PKCfrom the cytosol to the plasma membrane. Scale bar, 7 μm. (g) Diary plots and population bar charts showing PdBu-induced inhibition of CaV2.2, CaV2.1 and CaV1.2 channels co-expressed with mCherry-CaMKII1–274,K42M-C1PKC. Data are means±s.e.m. (h) Schematic and confocal image showing constitutive membrane targeting of mCherry-CaMKII1–274,K42M-KRastail. Scale bar, 5 μm. (i) Constitutive inhibition of CaVchannels by mCherry-CaMKII1–274, K42M-KRastail. Same format as (c). Data are means±s.e.m,n=5 for each point. *P<0.05 compared with control data by two-tailed Student’s pairedt-test. Figure 3: Generalized method for generating CCBs from Ca V α 1 -binding proteins. ( a ) Schematic of Ca V channel α 1 subunit. Four homologous domains (I–IV) each with six transmembrane segments are joined by intracellular loops and bracketed by cytoplasmic N- and C termini. Various proteins bind Ca V α 1 intracellular domains including Ca V β, 14-3-3, CaM kinase II and calmodulin. ( b ) Confocal images showing PdBu-induced translocation of C1 PKCγ -mCherry-14-3-3 from the cytosol to the plasma membrane. Scale bar, 4 μm. ( c ) Diary plots and population bar charts showing PdBu-induced inhibition of Ca V 2.2, Ca V 2.1, and Ca V 1.2 channels co-expressed with C1 PKCγ -mCherry-14-3-3. Data are means±s.e.m. ( d ) Schematic and confocal image showing constitutive membrane targeting of mem-mCherry-14-3-3. Scale bar, 5 μm. ( e ) Population I–V curves showing constitutive inhibition by mem-mCherry-14-3-3 of Ca V 2.2 (black triangles, red triangles), Ca V 2.1 (black squares, red squares) and Ca V 1.2 (black circles, red circles) channels. Data are means±s.e.m, n =5 for each point. * P <0.05 compared with control data by two-tailed Student’s paired t -test. ( f ) PdBu-induced translocation of mCherry-CaMKII 1–274,K42M -C1 PKC from the cytosol to the plasma membrane. Scale bar, 7 μm. ( g ) Diary plots and population bar charts showing PdBu-induced inhibition of Ca V 2.2, Ca V 2.1 and Ca V 1.2 channels co-expressed with mCherry-CaMKII 1–274,K42M -C1 PKC . Data are means±s.e.m. ( h ) Schematic and confocal image showing constitutive membrane targeting of mCherry-CaMKII 1–274,K42M -KRas tail . Scale bar, 5 μm. ( i ) Constitutive inhibition of Ca V channels by mCherry-CaMKII 1–274, K42M -KRas tail . Same format as ( c ). Data are means±s.e.m, n =5 for each point. * P <0.05 compared with control data by two-tailed Student’s paired t -test. Full size image We next considered whether we could convert Ca 2+ -calmodulin-dependent protein kinase II (CaMKII) into a CCB. CaMKII has been found to constitutively bind Ca V 1.2 (ref. 29 ) and Ca V 2.1 (ref. 30 ) channels, respectively. CaMKII bound to Ca V 1.2 C terminus was found necessary for Ca 2+ -dependent facilitation of I Ca (ref. 29 ). Further, CaMKII binding to Ca V 2.1 C terminus slows channel inactivation kinetics and regulates short-term synaptic plasticity in neurons [30] . CaMKII holo-enzyme is a multimer of 12 monomeric subunits [35] . Each monomer (475 amino acids) has three distinct domains: an N-terminal catalytic domain (residues 1–274) that mediates kinase activity, a central regulatory domain (residues 275–314) that exerts basal auto-inhibitory control of the kinase domain and an association domain (residues 315–475) that mediates subunit assembly. The catalytic domain of CaMKII mediates binding to Ca V 1.2 channels [29] . To assess the possibility of converting CaMKII into a CCB we fused either C1 PKCγ or the polybasic membrane-targeting tail from K-Ras to the C terminus of CaMKII catalytic domain (residues 1–274). We also introduced a K42M point mutation that renders the kinase catalytically dead [35] . CaMKII [1–274,K42M] -C1 PKC inducibly translocated to the membrane ( Fig. 3f ) and inhibited Ca V 2.2 and Ca V 1.2 channels in response to PdBu ( Fig. 3g ). Surprisingly, Ca V 2.1 channels were not inhibited by membrane-translocated CaMKII [1–274,K42M] -C1 PKC ( Fig. 3g , middle). By contrast, CaMKII [1–274,K42M] -KRas tail was constitutively associated with the plasma membrane ( Fig. 3h ), and caused a deep inhibition of all three Ca V channels ( Fig. 3i ). Beyond providing an additional proof of the principle for generating novel genetically encoded CCBs, these results suggest that recombinant Ca V 2.2 channels may also bind CaMKII. The discrepancy in Ca V 2.1 sensitivity to CaMKII [1–274,K42M] -C1 PKC and CaMKII [1–274,K42M] -KRas tail suggests that inhibition by the CaMKII-based inhibitor in this channel may be kinetically slow such that it is only apparent with the constitutive CCB. Finally, we explored the feasibility of using CaM to create a genetically encoded CCB. CaM is known to bind Ca V 1 and Ca V 2 channels and mediates their regulation by Ca 2+ ions. We generated mCherry-CaM-C1 PKC , which displayed basal cytosolic localization but was translocated to the plasma membrane with PdBu ( Fig. 4a ). As the endogenous CaM concentration is relatively high, the efficacy of CaM-based CCBs would be expected to depend critically on how effectively they displace endogenous CaM from the channels. We used Ca 2+ -dependent inactivation (CDI) of Ca V 1.2 channels as a biosensor to gain insights into how effectively C1 PKC -tagged wt and mutant CaM displaced endogenous CaM. When co-expressed with mCherry-CaM-C1 PKC , recombinant Ca V 1.2 channels (α 1C +β 2a ) displayed Ba 2+ currents that showed a slow monotonic voltage-dependent inactivation ( Fig. 4b ). With Ca 2+ as charge carrier, the same channels exhibited a fast and deep decrease in current amplitude with the kinetic signature of CDI ( Fig. 4b ). When co-expressed with a mutant mCherry-CaM 1234 -C1 PKC with all four EF hands mutated so they no longer bind Ca 2+ , Ca V 1.2 channels displayed Ca 2+ currents in which CDI was virtually eliminated ( Fig. 4b ). This result indicates that the over-expressed mCherry-CaM 1234 -C1 PKC effectively out-competes endogenous CaM for binding to Ca V 1.2, and further demonstrates that the tags do not interfere with CaM binding to Ca V channels. We found Ca V 2.2 channels co-expressed with mCherry-CaM 1234 -C1 PKC were rapidly inhibited by PdBu ( Fig. 4c ). Surprisingly, both Ca V 2.1 and Ca V 1.2 co-expressed with mCherry-CaM 1234 -C1 PKC were unaffected by PdBu ( Fig. 4c ). As CaM binds to all three channels [32] , [33] , [36] , [37] , these results suggest that the mere existence of a binding site for a cytosolic protein on the channel may not be sufficient to generate an inducible CCB in all cases. Another possibility is that potential inhibition of Ca V 2.1 and Ca V 1.2 induced by membrane-targeting mCherry-CaM 1234 -C1 PKC is kinetically slow such that it does not occur during the 5–10 min time course of our electrophysiological assay. 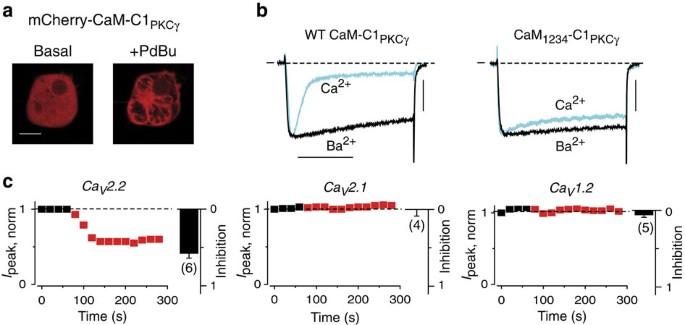Figure 4: A CaM-based PdBu-inducible CCB selectively inhibits CaV2.2 channel currents. (a) Confocal image showing PdBu-induced translocation of mCherry-CaM-C1PKCfrom cytosol to the plasma membrane in a transfected HEK 293 cell. Scale bar, 5 μm. (b) The C1PKCtag does not affect the functional interaction of CaM or CaM1234with CaV1.2. Scale bar, 0.5 nA, 10 ms. (c) Diary plots and population bar charts showing PdBu-induced effects of CaV2.2, CaV2.1 and CaV1.2 channels co-expressed with mCherry-CaM-C1PKC. Data are means±s.e.m. Figure 4: A CaM-based PdBu-inducible CCB selectively inhibits Ca V 2.2 channel currents. ( a ) Confocal image showing PdBu-induced translocation of mCherry-CaM-C1 PKC from cytosol to the plasma membrane in a transfected HEK 293 cell. Scale bar, 5 μm. ( b ) The C1 PKC tag does not affect the functional interaction of CaM or CaM 1234 with Ca V 1.2. Scale bar, 0.5 nA, 10 ms. ( c ) Diary plots and population bar charts showing PdBu-induced effects of Ca V 2.2, Ca V 2.1 and Ca V 1.2 channels co-expressed with mCherry-CaM-C1 PKC . Data are means±s.e.m. Full size image Overall, these data demonstrate that diverse intracellular proteins interacting with Ca V 1/Ca V 2 channels can be converted into constitutive or inducible CCBs with distinctive potency and/or selectivity. We have termed this general method Channel Inactivation induced by Membrane-tethering of an associated Protein (ChIMP). The acronym is apropos given the imagery of closing a channel pore by the induced ‘swinging’ of an associated protein from the cytoplasm to the plasma membrane ( Fig. 2a ). Effectiveness of 14-3-3-based CCB on native Ca V channels The results to this point have tested the efficacy of genetically encoded CCBs on recombinant Ca V channels reconstituted in HEK 293 cells. As native Ca V channels are typically associated with macromolecular complexes and have a more complicated nano-enviroment than recombinant channels in heterologous cells, it was important to verify that the genetically engineered CCBs were effective against native Ca V channels. We first examined the impact of mem-mCherry-14-3-3ε on Ca V channels recorded from primary cultures of murine dorsal root ganglion (DRG) neurons. DRG neurons express multiple Ca V 1/Ca V 2 channel currents [38] . We used adenoviral vectors to express either mCherry-14-3-3 or mem-mCherry-14-3-3 ( Fig. 5a ) in cultured DRG neurons. Cells expressing mCherry-14-3-3 displayed an I – V relationship that was indistinguishable from that obtained with control uninfected neurons ( Fig. 5b , left; I peak at 0 mV=57.2±9.9 pA/pF, n =6 for control neurons, I peak =62.0±19.6 pA/pF, n =6 for mCherry-14-3-3-expressing neurons). By contrast, expression of mem-mCherry-14-3-3ε in DRG neurons markedly suppressed endogenous I Ba within 24 h of adenoviral infection ( Fig. 5b , right; I peak =6.3±1.5 pA/pF, n =6 for mem-mCherry-14-3-3-expressing neurons, P <0.05 compared with control using unpaired t -test). We obtained similar results for nerve growth factor (NGF)-differentiated rat pheochromocytoma (PC12) cells ( Fig. 5c ), which contain Ca V 2.2 and Ca V 1.2 channels that trigger exocytosis [39] . These results demonstrate that genetically engineered CCBs developed according to the ChIMP principle are also effective against native Ca V 1/Ca V 2 channels despite their more elaborate nano-environment. 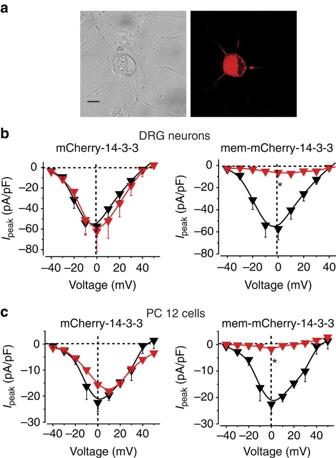Figure 5: Constitutive inhibition of endogenousICain native cells with 14-3-3-based CCBs. (a) Greyscale and fluorescence image of DRG neuron expressing mem-mCherry-14-3-3. Scale bar, 5 μm. (b) PopulationI–Vcurves in DRG neurons. Uninfected neurons (black triangles) compared with neurons expressing either mCherry-14-3-3 (left) or mem-mCherry-14-3-3 (right),n=6 for each point. (c) PopulationI–Vcurves in differentiated PC12 cells, same format as (b),n=5 for each point. *P<0.05 compared with control data by two-tailed Student’s pairedt-test. Figure 5: Constitutive inhibition of endogenous I Ca in native cells with 14-3-3-based CCBs. ( a ) Greyscale and fluorescence image of DRG neuron expressing mem-mCherry-14-3-3. Scale bar, 5 μm. ( b ) Population I–V curves in DRG neurons. Uninfected neurons (black triangles) compared with neurons expressing either mCherry-14-3-3 ( left ) or mem-mCherry-14-3-3 ( right ), n =6 for each point. ( c ) Population I–V curves in differentiated PC12 cells, same format as ( b ), n =5 for each point. * P <0.05 compared with control data by two-tailed Student’s paired t -test. Full size image Potential use of ChIMP to discover small-molecule CCBs The results so far suggest the general principle that the discovery process for new CCBs may be decomposed into two parts: first, finding a molecule that binds an appropriate α 1 -subunit cytoplasmic region (a ‘handle’) and second, a transduction step involving the anchoring of the ‘handle’ molecule to the plasma membrane. We next considered two ancillary issues. First, whether the ‘handle’ could be a small molecule rather than a protein as we have so far demonstrated. If so, the ChIMP method could potentially be extended to small-molecule drug discovery. Second, whether it would be possible to develop a method to systematically identify which areas in α 1 cytoplasmic regions are appropriate target-binding sites that are permissive for regulated closure of the channel pore. To concurrently address these two issues, we adapted a heterodimerization strategy that relies on the ability of the small-molecule rapamycin to simultaneously bind two proteins, FK506-binding protein (FKBP) and a fragment of the mammalian target of rapamycin (FRB), respectively [40] . We inserted FKBP (one insert per channel) at four different positions within Ca V 1.2 α 1C subunit intracellular regions (N terminus, I–II loop, and at proximal and distal positions in the C terminus) ( Fig. 6a ). All these constructs expressed currents when co-expressed with β 2a and a constitutively membrane-targeted FRB (LDR) in HEK 293 cells [18] , [41] . Rapamycin (1 μM) caused a rapid inhibition of I Ba in channels with FKBP inserted into the C terminus ( Fig. 6d,e ). By contrast, channels with FKBP inserted at the N terminus and in the distal I–II loop, respectively, did not display rapamycin-induced decrease in current ( Fig. 6b,c ). Neither of the two C terminus FKBP-fused channels responded to rapamycin in the absence of LDR ( Supplementary Fig. S7 ). These findings offer a critical proof-of-concept that the ChIMP approach can potentially be used to discover new CCBs by using high-throughput screening to find molecules that bind appropriate ‘handle sites’ in Ca V α 1 -subunits, and conjugating them to a membrane-targeting module. A major challenge that needs to be overcome to realize this possibility is developing sensitive high-throughput screens to identify small molecules that bind intracellular domains of Ca V channels. One possibility is to use purified tagged Ca V α 1 intracellular loops to probe small-molecule microarrays [42] , [43] . 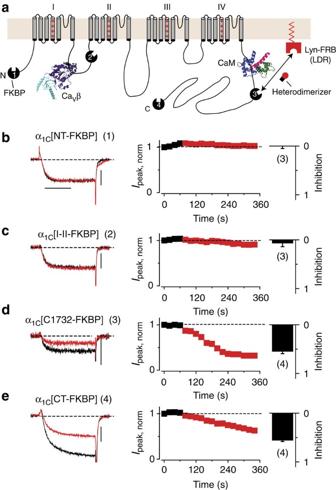Figure 6: Principle for developing novel small-molecule CCBs demonstrated using heterodimerization strategy. (a) Insertion of FKBP into selected regions of α1Cintracellular loops/termini. (b–e) Impact of rapamycin onIBafrom distinct FKBP-fused α1Cconstructs co-transfected with LDR. Scale bar, 400 pA, 10 ms. Figure 6: Principle for developing novel small-molecule CCBs demonstrated using heterodimerization strategy. ( a ) Insertion of FKBP into selected regions of α 1C intracellular loops/termini. ( b – e ) Impact of rapamycin on I Ba from distinct FKBP-fused α 1C constructs co-transfected with LDR. Scale bar, 400 pA, 10 ms. Full size image In this work we report the discovery that diverse proteins/molecules that bind distinct sites in intracellular loops of Ca V 1/Ca V 2 channels can be used as ‘handles’ to inhibit I Ca through their controlled anchoring to the plasma membrane. This new insight paves the way for developing customized CCBs with selectivity for distinct Ca V 1/Ca V 2 channels based on the identity of the pore-forming α 1 -subunit, the auxiliary Ca V β or other associated cytoplasmic proteins. Genetically encoded CCBs are potentially desirable because they can be expressed in a geographically restricted fashion thereby eliminating off-target effects that may confound small-molecule drug therapy [2] , [10] . Furthermore, genetically encoded CCBs can be engineered to block molecularly identical Ca V channels with sub-cellular specificity. For example, a caveolae-targeted Rem has been shown to selectively inhibit caveolae-localized Ca V 1.2 channels in heart cells while sparing dyadic Ca V 1.2 channels that trigger muscle contraction [14] . As caveolae-localized Ca V 1.2 channels are hypothesized to selectively signal to pathological cardiac hypertrophy, it is proposed that caveolae-specific Ca V 1.2 channel inhibitors could be an effective therapy for adverse remodelling of the heart [14] . RGK proteins have so far been used in proof-of-concept experiments to demonstrate the utility of genetically encoded CCBs [10] , [14] . However, the potential clinical use of RGKs is complicated by their broad biological effects, diverse binding partners and lack of specificity and controllability [11] . This work introduces ChIMP as a generalized method for developing novel genetically encoded CCBs with distinct potency, selectivity and kinetics. A caveat for the work is that the CCBs we have generated so far are derived from naturally occurring proteins that also have their own specific functions and binding partners in cells. Nevertheless, the general insights obtained from developing these proteins can now be potentially coupled with new technologies for evolving protein molecules that bind to target sites with high specificity, such as DARPins [44] and intrabodies [45] , to develop highly selective Ca V 1/Ca V 2 channel blockers. Another aspect of the ChIMP technology that can be greatly improved relates to the method for inducing membrane targeting of the ‘handle’ protein. Here we used PdBu and rapamycin-mediated heterodimerization as convenient tools to demonstrate proof-of-concept of the ChIMP method. However, PdBu activates endogenous protein kinase C, and rapamycin associates with endogenous FKBP and mammalian target of rapamycin (mTOR), a protein kinase involved in cell proliferation, growth and survival. Hence, these two agents may be inappropriate for potential in vivo applications. Recently, several genetically encoded dimerizers based on plant photoreceptors that permit light-regulated, reversible protein heterodimerization have been developed [46] , [47] , [48] . Marriage of light-regulated heterodimerization with ChIMP could provide a powerful general method for optogenetic control of Ca V channels and is an exciting prospect for future experiments. We previously reported that Rem, which normally constitutively targets to the plasma membrane and inhibits Ca V channels, could be converted into a small-molecule-regulated inducible CCB by dynamically regulating its association with the plasma membrane [18] , [19] . However, it was unknown how targeting Rem to the membrane caused Ca V channel inhibition. This work supports a model where membrane-targeted Rem uses Ca V β as a bridge to alter the conformation of the I–II loop in a manner that closes the channel. This is an important new insight into the mechanism of action of RGKs, particularly in light of data that have raised questions about a role for RGK binding to Ca V β in the mechanism for Ca V channel inhibition [49] . More generally, regulation of channel gating by induced conformational changes in intracellular domains is a rather common phenomenon that occurs in many different ion channels. For example, cyclic nucleotides and Ca 2+ control the opening of cyclic nucleotide-gated (CNG) and large conductance K + (BK) channels, respectively, by binding to channel intracellular domains [50] , [51] . Moreover, engagement of cytoplamic domains with the plasma membrane through interaction with phosphoinositide lipids regulates the gating of ion channels such as the inward rectifier K + channel Kir2.2 (ref. 52 ) and TRPV1 (ref. 53 ). From this perspective, the ChIMP approach could provide important insights into how distinct intracellular domains link to channel gating in different ion channels. The major conceptual advance in this study is that diverse cytosolic proteins or small molecules that bind distinct sites in intracellular loops of Ca V 1/Ca V 2 channels can likewise be converted to constitutive or inducible Ca V channel inhibitors according to the mode of their anchoring to the plasma membrane. This is a non-trivial advance because it suggests a general method for developing novel genetically encoded blockers for many ion channel types. Ion channels are ubiquitous and essential to the biology of all cell types, and their dysfunction underlies many human diseases [54] . Selective ion channel modulators are highly sought after as therapeutics and research tools. However, there is a lack of specific modulators for many ion channel species. The ChIMP strategy may potentially be applied to develop novel blockers for a broad cohort of ion channels. A corollary benefit of the ChIMP approach is its potential to provide a robust functional readout as to whether individual proteins directly interact with intracellular domains of recombinant Ca V 1/Ca V 2 channels. In our study, we discovered for the first time that recombinant Ca V 1.2 binds 14-3-3 and that Ca V 2.2 binds CaMKII. A proteomic study of the Ca V 2 channel nano-environment in mammalian brain indicates these channels are associated with a protein network gathered from a pool of ~200 proteins with distinct abundance and preference for Ca V 2.1–Ca V 2.3 subtypes [55] . Our studies suggest how Ca V 1/Ca V 2 channels may be used as a biosensor to validate some of these putative protein interactions. cDNA cloning To generate fluorescent-protein-tagged constructs, cyan or yellow fluorescent protein (CFP or YFP) was amplified using PCR and cloned into pcDNA4.1 (Invitrogen) using Kpn I and BamH I sites. CFP–Rem 1–265 –C1 PKCγ and CFP–Rem 1–250 –C1 PKCγ were generated by using overlap extension PCR to fuse residues 26–89 of mouse PKCγ to the C terminus of Rem 1–265 and Rem 1–250 , respectively. The fusion product was subsequently cloned downstream of CFP using BamH I and EcoR I sites. To create C1 PKCγ -Rem 78–265 –CFP, C1 PKCγ was cloned into pcDNA4.1 (Invitrogen) using Kpn I and BamH I sites. Rem 78–265 and CFP were subsequently amplified and cloned downstream of C1 PKCγ using BamH I/ EcoR I and EcoR I/ Xba I sites, respectively. C1 PKCγ -YFP-Rem 1–265 was produced by first using overlap extension PCR to fuse C1 PKCγ to the N terminus of YFP. The resulting fusion product was cloned upstream of Rem 1–265 using Kpn I and BamH I sites. CFP-β 3 -C1 PKCγ was generated by using overlap extension PCR to fuse C1 PKCγ to the C terminus of β 3 . The fusion product was then cloned downstream of CFP using BamH I and EcoR I sites. To generate C1 PKCγ -mcherry-14-3-3, we used overlap extension PCR to fuse C1 PKCγ to the N terminus of mCherry. The fusion product was cloned into pcDNA4.1 (Invitrogen) using Kpn I and BamH I sites. 14-3-3 was PCR amplified and cloned downstream of mcherry using BamH I and Xho I sites. To create mcherry-CaMKII 1–274K42M -C1 PKCγ , we used overlap extension PCR to fuse C1 PKCγ to the C terminus of CaMKII 1–274 . The fusion product was cloned into pcDNA4.1 (Invitrogen) using BamH I and Xho I sites sites. mcherry was PCR-amplified and cloned upstream using Kpn I and BamH I sites. Point mutation in mcherry-CaMKII 1–274K42M -C1 PKCγ was introduced using the QuikChange Site-Directed Mutagenesis Kit (Stratagene). To generate FKBP-fused α 1C constructs, we used overlap extension PCR to fuse YFP to the C terminus of α 1C . The fusion product was cloned into pcDNA3.1 (Invitrogen) using Kpn I and Xba I sites. FKBP was inserted into distinct regions of α 1C intracellular loops using In-fusion Cloning Kit (Clontech). All PCR products were verified by sequencing. Cell culture and transfection Low-passage-number HEK 293 cells were maintained in DMEM supplemented with 10% FBS and 100 μg ml −1 penicillin–streptomycin. For electrophysiology and flow cytometry experiments, HEK 293 cells cultured in 6-cm tissue culture dishes were transiently transfected with Ca V 1/Ca V 2 α 1 (6 μg), β 3 (6 μg), T antigen (2 μg) and the appropriate GEMIICC construct (4 μg), using the calcium phosphate precipitation method. Cells were washed with PBS 5–8 h after transfection and maintained in supplemented DMEM. For confocal microscopy experiments, transfected HEK 293 cells were replated onto fibronectin-coated culture dishes with No. 0 glass coverslip bottoms (MaTek). For electrophysiology experiments cells were replated onto fibronectin-coated glass coverslips 24 h after transfection. Murine dorsal root ganglion (DRG) neurons were kindly provided by the laboratory of Dr Joachim Scholz (Columbia University). DRG neurons were maintained in 96.5 ml Neurobasal A medium supplemented with 2 ml B-27, 100 μg ml −1 Pen/strep, 0.5 ml L -glutamine, 50 ng ml −1 NGF, 2 ng ml −1 GDNF and 10 μM Ara-C. For electrophysiology experiments, DRG neurons cultured in 2-cm tissue culture dishes were infected with the appropriate adenovirus. Undifferentiated PC12 cells were maintained in RPMI supplemented with 10% horse serum, 5% FBS and 100 μg ml −1 penicillin–streptomycin. Differentiated PC12 cells were maintained in RPMI supplemented with 1% horse serum. NGF (50 ng ml −1 ) was added to media just prior to use. For electrophysiology experiments, PC12 cells cultured in 6-cm tissue culture dishes were infected with the appropriate adenovirus. Electrophysiology Whole-cell recordings of HEK cells were conducted 48–72 h after transfection using an EPC—8 or EPC—10 patch clamp amplifier (HEKA Electronics) controlled by PULSE software (HEKA). Micropipettes were fashioned from 1.5-mm thin-walled glass with filament (WPI Instruments) and filled with internal solution containing (in mM): 135 caesium methanesulphonate (CsMeSO 3 ), 5 CsCl, 5 EGTA, 1 MgCl 2 , 4 MgATP (added fresh) and 10 HEPES (pH 7.3). Series resistance was typically between 1.5–2 MΩ. There was no electronic series resistance compensation. External solution contained (in mM): 140 tetraethylammonium—MeSO 3 , 5 BaCl 2 , and 10 HEPES (pH 7.3). Whole-cell I – V curves were generated from a family of step depolarizations (−40 to +100 mV from a holding potential of −90 mV). Currents were sampled at 25 kHz and filtered at 5 or 10 kHz. Traces were acquired at a repetition interval of 6 s. Leak and capacitive currents were subtracted using a P/8 protocol. Whole-cell recordings of DRG and PC12 cells were conducted 24–48 h after infection. HEK cell internal solution was used for both DRG and PC12 cells. HEK cell external solution was used for PC12 cells. HEK cell external solution with 0.5 μM TTX was used for DRG neurons. Confocal microscopy Static images of CFP–Rem 1–265 -C1 PKCγ , CFP-β 3 -C1 PKCγ , and mcherry-C1 PKCγ -14-3-3 constructs were observed using a Leica TCS SPL AOBS MP Confocal microscope system and a × 40 oil objective (HCX PL APO 1.25–0.75 NA). HEK 293 cells expressing CFP, YFP and mCherry fusion proteins were imaged using the 458-, 514- and 543-nm Argon laser line, respectively, for excitation. Data and statistical analyses Data were analysed off-line using PulseFit (HEKA), Microsoft Excel and Origin software. Statistical analyses were performed in Origin using built-in functions. Statistically significant differences between means ( P <0.05) were determined using Student’s t -test for comparisons between two groups or one-way ANOVA followed by pairwise means comparisons using Bonferroni test for multiple groups. Data are presented as means±s.e.m. How to cite this article: Yang, T. et al. Bio-inspired voltage-dependent calcium channel blockers. Nat. Commun. 4:2540 doi: 10.1038/ncomms3540 (2013).